Hydrogen bond rotations as a uniform structural tool for analyzing protein architecture Proteins fold into three-dimensional structures, which determine their diverse functions. The conformation of the backbone of each structure is locally at each C α effectively described by conformational angles resulting in Ramachandran plots. These, however, do not describe the conformations around hydrogen bonds, which can be non-local along the backbone and are of major importance for protein structure. Here, we introduce the spatial rotation between hydrogen bonded peptide planes as a new descriptor for protein structure locally around a hydrogen bond. Strikingly, this rotational descriptor sampled over high-quality structures from the protein data base (PDB) concentrates into 30 localized clusters, some of which correlate to the common secondary structures and others to more special motifs, yet generally providing a unifying systematic classification of local structure around protein hydrogen bonds. It further provides a uniform vocabulary for comparison of protein structure near hydrogen bonds even between bonds in different proteins without alignment. A hydrogen bond [1] forms between an electronegative atom (the acceptor) and a hydrogen atom covalently bound to another electronegative atom (the donor). Hydrogen bonds are of key importance in determining and fine-tuning molecular structure, interaction, function [2] and specificity of molecular recognition [3] . It is widely recognized that the function of a protein is intimately linked to the three-dimensional (3D) structure of its native folded state. Besides polypeptide assembly through covalent bonds, the structure is determined and stabilized by van der Waals interactions, hydrophobic packing, hydrogen bonds and ionic interactions. As hydrogen bonds are readily broken and reformed, they determine alternative conformations, and hence are also important for conformational changes of proteins. Dihedral angles specify the backbone conformation of proteins by providing a complete 2D description of the progression from one peptide unit to the next along the backbone, as displayed in the well-known Ramachandran plots [4] . However, dihedral angles are not reliable when considering relative configurations, which are separated far apart along the backbone. As the geometric phase space of hydrogen bonds has large dimension a priori , 3D and 4D simplifications have captured only part of their geometry [5] , [6] . Here, we introduce a systematic 3D descriptor of main chain hydrogen bond geometry by assigning to each hydrogen bond between backbone C=O and N–H atoms a spatial rotation, which is evidently independent of the overall spatial orientation of the protein just as for dihedral angles. The rotation is simply obtained as follows: First, rotate the entire protein, such that the donor peptide unit is aligned with the standard coordinate axes; the subsequent rotation from this standard location of the donor to the acceptor is the 3D descriptor of the hydrogen bond. As any rotation is given by a rotation axis and degree of rotation, it can be plotted in 3D space as a vector along the rotation axis of length equal to the degree of rotation. Hence all vectors in 3D space of length at most π describe all rotations. Rotations can thus be displayed by semi-transparent 2D projections on the page to graphically represent the geometry of main chain hydrogen bonds, akin to Ramachandran plots of dihedral angles for backbone geometry. Using a set of high-quality structures culled from the PDB [7] to probe the conformational space, we measure the rotations for the totality of hydrogen bonds (1.16 M hydrogen bonds) from all these structures and find, amazingly, that all the rotations concentrate into 30 well-defined clusters, which together comprise just over 32% of the volume of rotational space. In fact, 93.4% of all the rotations are contained in the seven biggest clusters occupying just under 20% of the volume of rotational space. This is particularly striking, as we find that fully 95% of the volume of rotational space is accessible when describing atoms as rigid spheres, whereas still 50% is available when modelling the hydrogen bonding of peptides with Density Functional Theory (DFT), accepting all bonds of at least 0.1 eV hydrogen bond strength. By analyzing the resulting data, we conclude that this rotation descriptor alone determines the relative configurations of the two peptide planes involved in the hydrogen bond, with one exception, which is explained in detail below. Our clusters correlate with well-known patterns such as α, 3 10 and π-helices, parallel and antiparallel β -structures, and further provide a collection of motifs found in random coil and turn elements of protein structure. All of this is obtained from our new systematic uniform viewpoint of rotations associated to backbone hydrogen bonds. In this way, the rotational descriptor provides a uniform viewpoint on local structural motifs around main chain hydrogen bonds in proteins. Practically speaking, as each such cluster displays specific structural characteristics, the associated classification of hydrogen bond geometry is useful in studying specific protein function and conformational changes. It further gives a novel vocabulary and a quantitative measure by which one can compare local configurations around hydrogen bonds within each structural element of a protein as well as between such, and even for hydrogen bonds from different proteins without requiring alignment. The rotational descriptor of main chain hydrogen bonds We associate a triple of orthogonal unit vectors (that originated in earlier work [8] ) to the i th peptide unit P i along the backbone by using only main chain coordinates. The first vector is the unit vector from the centre of the carbon atom C to the centre of the nitrogen atom N in the i th peptide bond. The second vector is obtained by rotating the first vector 90° towards the oxygen atom O in the same peptide plane, and the last vector is the cross-product of the two first ( Fig. 1a and Methods). For each i , there is a unique rotation , which brings the unit vectors parallel to the x , y and z axes to the triple associated to the i th peptide unit P i . 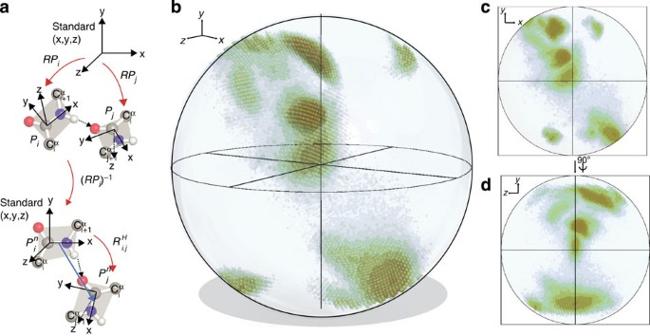Figure 1: Density plot of distribution of all hydrogen bond rotations in PDB-HQ60. (a) Hydrogen bond from peptide unitsPito peptide unitPj, where the locations of the backbone atoms, Ciand Ni+1(, Cjand Nj+1) determine a rotation. Rotation of both peptide units by the inverse ofbringsPiin standard position,andPjto a new positionand the rotation bringingtois the rotationassociated to the hydrogen bond. The blue arrow from the center of mass oftois the translation associated to the hydrogen bond. (b) 3D rendering of the total distribution coloured by density. (c) Orthoscopic projection of the density plot in thex–yplane. (d) Orthoscopic projection of the density plot in thex–zplane. To a hydrogen bond from donor peptide unit P i to acceptor peptide unit P j , we assign the rotational descriptor Figure 1: Density plot of distribution of all hydrogen bond rotations in PDB-HQ60. ( a ) Hydrogen bond from peptide units P i to peptide unit P j , where the locations of the backbone atoms , C i and N i +1 ( , C j and N j +1 ) determine a rotation . Rotation of both peptide units by the inverse of brings P i in standard position, and P j to a new position and the rotation bringing to is the rotation associated to the hydrogen bond. The blue arrow from the center of mass of to is the translation associated to the hydrogen bond. ( b ) 3D rendering of the total distribution coloured by density. ( c ) Orthoscopic projection of the density plot in the x – y plane. ( d ) Orthoscopic projection of the density plot in the x – z plane. Full size image ( Fig. 1a and Methods). According to Euler’s rotation theorem [9] , a rotation is determined by an axis, that is, a vector of unit length, together with an angle θ (in radians) of rotation around it. We plot such a rotation as a point in 3D space conveniently imagined as a sphere of radius π representing all rotations, so-called rotational space plots ( Fig. 1b , where we stress that antipodal points on the surface sphere of radius π represent the same rotation). This descriptor of a hydrogen bond together with the translation vector rotated by (blue arrow, Fig. 1a ) from the center of mass of the donor peptide unit to the center of mass of the acceptor peptide unit completely describes the relative positions of a pair of peptide units. However, it is only the rotational part studied here that exhibits the characteristic clustering; in fact, the rotation substantially determines the translation for main chain hydrogen bonds (see discussion below), and hence our 3D rotational descriptor likewise determines the geometry of the hydrogen bond. Specification of the protein databases We study three basic classes of databases. Two are derived from PISCES [10] runs with PDB [7] on 12 March 2012: which are taken at 15, 30, 60 and 95% sequence identity. The third set is the CATH [11] v.4.0.0 library at the levels CATHS, CATHSO, CATHSOL together with ‘CATH’, a set identified by the CATH developers at the CATH—CATHS level of their database. See Supplementary Note 1 for further specification of the databases. A Dictionary of the Secondary Structure of Proteins (DSSP) [12] hydrogen bond is accepted provided [13] furthermore that: We remark that our condition for accepting a hydrogen bond depends on the location of the H atom at the amide end in each hydrogen-bonded peptide unit. Please see Supplementary Note 2 for a discussion of the determination of the H atom locations. Our reference library is HQ60, namely, high-quality data at 60% sequence identity containing 1.16 M hydrogen bonds. A density plot of the raw data ( Fig. 1b–d and Supplementary Fig. 1 ) reveals remarkably that the rotations cluster and concentrate in a relatively small volume of rotational space. Cluster determination Several runs of the clustering algorithm detailed under Methods were performed. A first run of the clustering algorithm using all the data together resulted in 14 clusters comprising >99.99% of all the data. Inspection of most of these clusters revealed that the mode box was composed primarily of hydrogen bonds of one fixed length along the backbone. Also, an examination of the translation vectors for these 14 clusters pointed to further limited sub-clustering. For this reason, we refined the analysis by making a separate clustering for each signed difference Δ from donor to acceptor. Precisely, if the hydrogen bond is from donor peptide unit P i to acceptor peptide unit P j , then Δ= j − i if i < j and otherwise Δ= j − i −1 ( Fig. 2 ). 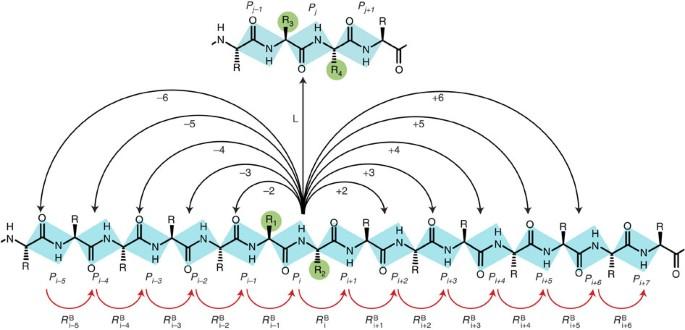Figure 2: Indexing conventions of hydrogen bonds. The flanking residuesR1,R2,R3andR4around the hydrogen bond fromPitoPj, the signed length Δ of hydrogen bonds along the backbone and the long-rangeL-group of hydrogen bonds corresponding to |Δ|>6. The rotations along the backboneindicate the rotations from theith peptide unitPito the followingPi+1. Figure 2: Indexing conventions of hydrogen bonds. The flanking residues R 1 , R 2 , R 3 and R 4 around the hydrogen bond from P i to P j , the signed length Δ of hydrogen bonds along the backbone and the long-range L -group of hydrogen bonds corresponding to |Δ|>6. The rotations along the backbone indicate the rotations from the i th peptide unit P i to the following P i +1 . Full size image For |Δ|>6, we did not find any differences in the clustering results, and thus all data with |Δ|>6 were combined into a ‘long-range’ group. Thus, we considered separately Δ=−2, Δ=2, Δ=−3, Δ=3, Δ=−4, Δ=4, Δ=−5, Δ=5, Δ=−6, Δ=6 and |Δ|>6. The clustering algorithm discussed above was run for each of these length categories and resulted in 29 clusters. For each of these clusters, the corresponding translation vectors were considered, and except for the main cluster with Δ=−3, the translations did not point to any further sub-clustering. For the main cluster with Δ=−3, there was a clear division into two sub-clusters as illustrated in Supplementary Fig. 2 . In this way, we ended up with the total of 30 clusters listed in Table 1 and plotted in Fig. 3 . The notation for the clusters with |Δ|≤6 is Table 1 Characteristics of the 30 clusters in rotational space based on PDB-HQ60. 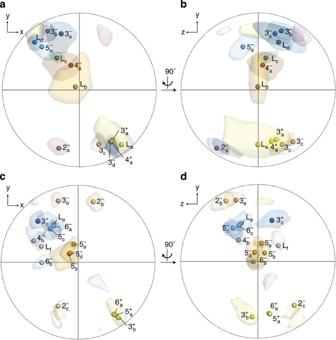Figure 3: Plots of the 30 clusters in rotational space. (a) and (b) are orthoscopic projection plots of the 15 biggest clusters along thezandxaxis. (c) and (d) are orthoscopic projection plots of the 15 smallest clusters along thezandxaxis. Full size table Figure 3: Plots of the 30 clusters in rotational space. ( a ) and ( b ) are orthoscopic projection plots of the 15 biggest clusters along the z and x axis. ( c ) and ( d ) are orthoscopic projection plots of the 15 smallest clusters along the z and x axis. Full size image where the subindex is an alpha-numeric enumerator, indexing clusters according to decreasing size (measured in terms of data points in clusters) for a given value of Δ. For the clusters with |Δ|>6, we use the notation L a,b,c,… , where again the alpha-numeric enumerator indexes clusters according to decreasing size. We have further listed the volume (given in % of the total volume of rotational space), the average and maximal distance within a cluster to the mode and the average distance to the mode among the top 70% of the density. The latter being a measure for how peaked the cluster is with a small value, indicating a peaked distribution and a large value a flat distribution. We observe that even though cluster contains almost half of the hydrogen bonds, it only occupies a little <2.5% of the volume. It is the most peaked cluster, about two times more so than and 3.5 times more so than L a and L b , which are the other large clusters. We further observe that L a and L b have considerably larger volume than any other cluster. We see that , and L a have the largest possible maximal distance to the mode, namely π. We observe that 93.4% of the data are contained in the seven largest clusters , L a , L b , , , , , which together occupy just below 20% of the volume of rotational space. Supplementary Fig. 3 provides for each cluster a plot showing the maximal, minimal and average logarithmic density as a function of distance to the mode. This provides a more detailed description of how peaked the individual clusters are. In Fig. 4 we provide a sample structure for each of the 30 cluster, whose rotation belongs to the mode of the given cluster. 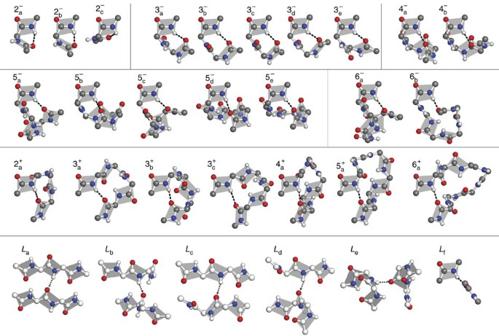Figure 4: Sample structure from the mode of each of the 30 clusters. Sample structure from the mode of each of the 30 clusters divided according to length along the backbone. Figure 4: Sample structure from the mode of each of the 30 clusters. Sample structure from the mode of each of the 30 clusters divided according to length along the backbone. Full size image The original 14 modes from the run with all hydrogen bond rotations together, independent of Δ can be found as the modes of the final clusters , , , , , , , , , , , L a , L b and L d . As can be seen, none of the original modes correspond to the Δ>0 length categories. This reflects the fact that the modes of Δ>0 clusters are all close to the modes of the long-range clusters L a ,…, L f . Clustering has also been analyzed using all of the above-mentioned data sets and the less stringent DSSP [12] definition of hydrogen bonds with substantially the same conclusions as with the high-quality PDB-based libraries in this paper. To further access the stability of the clusters under change of the clustering algorithm, we have also implemented the Mean shift clustering algorithm [14] , [15] , [16] , which similarly reproduces the same clustering with minor variations. Please see Supplementary Note 3 for a discussion of the selection of the clustering algorithms and Supplementary Note 4 and Supplementary Table 1 for a comprehensive comparison of all clustering runs. Hydrogen bonds clusters and Ramachandran plots To demonstrate that there, in general, are no relations between our 3D rotational descriptor of hydrogen bonds and the Ramachandran plots at the flanking C α , we have in Supplementary Fig. 4 plotted the Ramachandran plots for all the hydrogen bonds in a given cluster for each of the four locations indexed as indicated in Fig. 2 . None of the 15 biggest clusters exhibits a strong localization of any of the four Ramachandran plots. All large clusters and most of the small clusters have a broad spread of the flanking conformational angles. Hence our 3D rotational descriptor of hydrogen bonds is akin to the Ramachandran plots but is by no means determined by the flanking Ramachandran plots. Certain clusters do, however, have significantly higher density at certain conformational angles. The large cluster has a peak at the conformational angles of the 3 10 helix, at the α helix and L a and L b at the β -strand conformational angles. We also in part see this for some of the short-range clusters at certain of the positions R 1 ,…, R 4 , for example, for clusters , , , , , . It is, however, still clear that we do not even in these cases see a localized single cluster behaviour, except for the following very small clusters , , and . All of this fits well with the following analysis of the primary and secondary imprints of our clusters and the following correlation analysis between our clusters compared with known structural motives. Characterizing primary/secondary structure imprints To explore the primary/secondary propensities of the clusters, we evaluate the primary and secondary structure of the four residues of the donor and acceptor peptide units. The residues are annotated R 1 , R 2 , R 3 and R 4 as in Fig. 2 , where R 2 contains the donor amide and R 3 contains the donor carbonyl. The residue distribution for the clusters is plotted in the left column of Supplementary Fig. 5 . Clusters and have a 30% occurrence of Glycine at position R 1 = R 4 . and have a 70% occurrence of Glycine at position R 1 , whereas has a 65% occurrence of Glycine at R 4 . The cluster has 95% Proline at R 1 . These findings correspond closely to the known residue preferences for γ and β turns. Cluster has a 20–40% occurrence of Glycine at R 1 ,…, R 4 showing that this longer turn motif requires a Glycine to bend the backbone, with the position of the Glycine being less important. As we will observe below, , and have similar hydrogen bond rotational geometry, which is also reflected here by a shared preference for Glycine at R 1 of 60–95% and a preference for Leucine at R 2 of 20–35%. A few smaller preferences are observed for the +-clusters: has a preference for Glycine at R 1 of 40% and R 2 of 20%; has 25% Serine at R 2 ; and have a 20–30% preference for Aspartic acid at position R 2 . Long-range clusters L c , L e and L f show a 20–40% preference at R 1 or R 2 . In conclusion, the primary sequence of the clusters is only a weak signal characterized by Glycine, Proline and other amino acids that provide special backbone conformations. The primary sequence signatures of residue four-tuples were likewise investigated, but no highly occurring four-tuple patterns were observed (please see Supplementary Table 2 ). Next, we investigate the secondary structure patterns of the clusters by using the DSSP [12] annotation. DSSP annotates residues with seven secondary structure classes based on backbone geometry: H= α helix, B=residue in isolated beta-bridge, E=extended strand, participating in beta ladder, G=3-helix (3 10 helix), I=5-helix ( π helix), T=hydrogen bonded turn, S=bend, –=unclassified. The secondary structure preferences were plotted in Supplementary Fig. 5 (right column). Cluster is identified as unclassified by DSSP, whereas and are identified as S or T, respectively. Cluster shows a signal for 3 10 helix, α helix and turn on R 1−4 , which is in accordance with our ideal correlation of both 3 10 helix and beta-turn type I discussed below. Clusters and have the pattern T–T, whereas and are predisposed to TEET and correlated to beta turns. Cluster has a very strong HHHH signature, which corresponds to α helices consistent with the further analysis below. Cluster has a weaker DSSP predisposition, but shows preference of 40% for H at R 124 and 50% for T at R 12 . All 5 − and 6 − clusters have a strong preference for HH at R 34 . Cluster has ESSE pattern, whereas the remaining +-cluster and L-cluster have mainly E (beta) annotations. Turns and helixes For hydrogen bonds between peptide units in helixes and turns, we can compute the corresponding rotations as described under Methods. The natural distance measure between two rotations is the geodesic distance also recalled in the Method section. Table 2 lists the distances between the modes of clusters with backbone length Δ between −2 and −5 and the respective ideal structures ( Fig. 5 ). Thus, the modes of cluster and closely correspond to the ideal gamma turns ( Fig. 5a ). Cluster has its mode exactly at the ideal α helix, whereas the mode of cluster is close to the alpha turn I− α RU ( Fig. 5c ). Alpha turn IRS lies in , whereas the remaining alpha turns lie in . For length Δ=−5 clusters, the mode of is particularly close to the Schellman motif and also close to HB-AAAa. The modes of clusters , , are closets to the ideal π helix rotation and is closets to the Schellman motif. Pi turn HB-PgAA lies in cluster and HB-AAAA in ( Fig. 5d ). The cluster to which the exact ideal hydrogen bond rotation either belongs or is closest to, for each motif, is given in the last column of Supplementary Table 3 . Table 2 Distances between cluster modes and idealized gamma/beta/alpha/pi-turns. 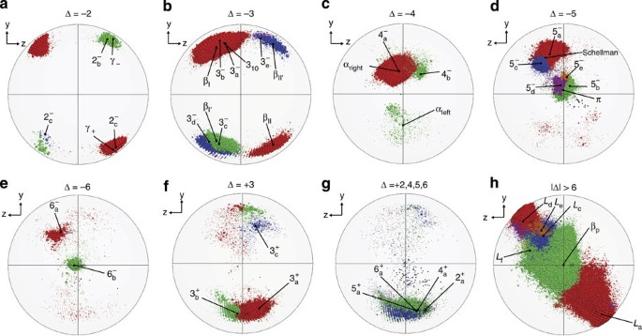Figure 5: Comparison between ideal motives and clusters. For each signed length Δ along the backbone, the clusters are plotted (in red, green, blue and orange) with indication of the mode location of the cluster together with the location of some of the ideal structures in rotational space:γ±for 2−,βI,βII,βI′,βII′for 3−,αright,αleftfor 4−, Schellman, π for 5−andβpforL. The lettersatohindicate the different length categories. Full size table Figure 5: Comparison between ideal motives and clusters. For each signed length Δ along the backbone, the clusters are plotted (in red, green, blue and orange) with indication of the mode location of the cluster together with the location of some of the ideal structures in rotational space: γ ± for 2 − , β I , β II , β I ′ , β II ′ for 3 − , α right , α left for 4 − , Schellman, π for 5 − and β p for L . The letters a to h indicate the different length categories. Full size image To further investigate the beta turns, we have for each of the five clusters ,…, calculated the occurrences of the eight turn types ( Supplementary Table 4 ). Using the conformational angles in Supplementary Table 3 , a turn belongs to a turn type [17] if three angles deviate <30° from the ideal values and the last deviates by at most 45°. From the Supplementary Table 4 , it appears that cluster is dominated by 3 10 helices and beta turn I, cluster by beta turn II, by beta turn I′, by beta turn II′, and cluster by beta turn VIa1 although this turn is found in and as well. The distances from the mode points of the clusters to the ideal structures confirm these findings ( Fig. 5b ). To estimate the proportion of the bonds in clusters , and , , , which are involved in helical patterns, we have computed the proportion of the bonds in the cluster, which are flanked by bonds from the same length category. As it appears from Supplementary Table 5 , 80% (of which 17.5% are at ends) of the bonds in are involved in α-helixes, 39.5% (of which 35.5% are at ends) in 3 10 helixes. The majority of bonds from and half of the bonds in and ~30% of the bonds from are involved in π-helices. Beta turns VIa2, VIb and VIII are special in the sense that the hydrogen bonds calculated from the backbone conformational angles assuming idealized geometry are not to be found in the data set of hydrogen bonds. A closer study reveals that indeed these turns do not conform to idealized geometry, and hence one can simply not compute their rotations using conformational angles. The rotational space distance between the hydrogen bond rotation and the rotation calculated from the backbone conformational angles as assuming idealized geometry (and cis conformation in peptide plane two for VIa2 and VIb) are of the order 1–3 in distance instead of the order 0.2 in distance when idealized geometry holds. This demonstrates further the utility of over rotational descriptor, which in this case is much more accurate than backbone conformational angles. Long-range clusters For long-range hydrogen bonds, we can of course not proceed in the same way as for turns and helixes, moving very long distances along the backbone. We proceed instead inductively as described under methods. Using the notation from the Method section, Table 3 list the distances between and with , one of the six mode points for the long-range clusters and is given by either (15), (16) or (17) (with the distance the same for the two parts of the latter). The table also considers the relations appropriate for the case of a parallel and antiparallel beta strand being part of a beta sheet. The relations then involve both of and . Table 3 Relation on mode point rotations for long-range clusters and extended β -strands. Full size table The mode of cluster L b is close to the ideal extended parallel beta strand. The modes of clusters L a and L d are both close to the ideal extended antiparallel case, and both have a rotation angle close to π. Clusters L c , L e and L f all have an intermediate rotation angle. The mode of cluster L c is close to solving both of (15) and (16), whereas the mode of cluster L e is close to solving the latter only ( Fig. 5h ). The mode of cluster L f seems unrelated to extended beta strands. Actually, L f is the only cluster for which the transformed mode of the mode point is closer to the mode point of another cluster than to itself for the two antiparallel transformations (being closer to the mode point of L c , the distances being 1.11 and 0.77 from the two first entries of Table 3 ). The mode of cluster L d is very close to solving the equations when a parallel and antiparallel beta strand are neighbours in an antiparallel fashion. The mode of cluster L a has the same property, whereas the mode of cluster L b fits the corresponding equations when the two strands are neighbours in a parallel fashion. Looking at the Ramachandran plots for all of the clusters in Supplementary Fig. 4 , we see that, apart from the extended parallel and antiparallel beta strands, each cluster contains hydrogen bonds not related to these structures. Please see Supplementary Fig. 6 and Supplementary Note 5 for further discussion of this point. Beta hairpins Hydrogen bonds from beta hairpins will by their very nature appear in several clusters. Take as an example a 2:2 hairpin, where the inner hyrogen bond of the loop is a Beta turn (3 − clusters) and the next hydrogen bond along the strand belongs to one of the 3 + clusters. Table 4 gives the number of potential beta hairpins of the form described under Methods in the various clusters and the cluster annotation of the next hydrogen bond along the beta strand. Among 2:2 hairpins, as defined above, more than half are found in the combination with the second largest group in the combination . There are a few cases of 4:4 and 5:5 hairpins giving rise to the combinations and . Hairpins involving the long-range clusters are primarily found in L a , namely in the combinations , , , and . The only exception is a small number of 2:4 hairpins in the combination . The existence of beta hairpins in , , , helps explain the proximity of the modes of these clusters and the mode of long-range cluster L a . Table 4 Probing for Beta hairpins in the various clusters. Full size table Accessible part of the rotational space To assess, from a steric viewpoint, which part of rotational space is available for hydrogen bonding, we performed the following computation: all atoms of two free peptide units were described as rigid spheres and a search of translations was made to identify if the hydrogen bond criterion from DSSP and condition (3) could be met without any overlap of the rigid spheres occurring for non-covalently bonded atoms. For each grid point (grid size 2π/81) inside the sphere of radius π, up to 21,952 different translations were tested against the hydrogen bond recognition criteria. If a translation resulting in an acceptable hydrogen bond was found, then the above test was performed. With these constraints, it was found that 95% of rotational space had at least one possible translation that resulted in a hydrogen bond ( Fig. 6c ). The observed high-density regions in rotational space are thus not a consequence of steric constraints alone. As the default restrained refinement of structures obtained by X-ray crystallography only includes a standard set of stereo-chemical restraints (covalent bonds, angles, dihedrals, planarities, chiralities, non-bonded), the just mentioned analysis further demonstrates that the observed clustering cannot be seen as a consequence of this refinement process either. 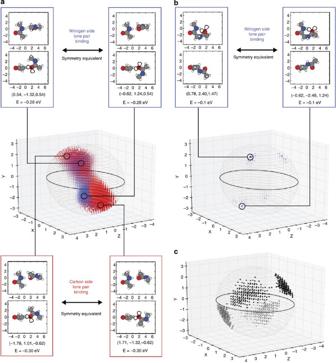Figure 6: DFT calculations for CH3–NH–CO–-CH3 dimer and CH3–NH–CO–CH2–NH–CO–CH3. (a) For each sampled point in rotational space, a sphere is plotted whose radius is proportional to the Boltzmann weight factor exp(−E/kT) of that point at room temperature with the normalization constant chosen such that points with 0.1 eV above the global minimum of −0.30 eV vanish. By this procedure, hydrogen bonds of at least 0.2 eV strength appear coloured in the figure and are found to comprise 32% of the entire volume of rotational space. Assessing the volume taken up by hydrogen bonds of at least 0.1 eV strength, one reaches 50% of the volume of rotational space.The most stable bonding class is that of the acceptor molecule binding through the O-lone pair, which is at the methyl side of the carbonyl (red spheres in the figure). The other significant bonding class is that of the acceptor molecule binding through the O-lone pair, which is at the amide side of the carbonyl (blue spheres in the figure). Both are doubly degenerate because of symmetry. (b) This plot is prepared just as (a) is, but here for two consecutive peptide units along the backbone, and only one bonding class (modulo symmetry) is identified. These two minima are recognized asγ+andγ−turns, respectively. (c) Plot of the volume in rotational space (black points) with prohibitive steric overlap of rigid atomic spheres. The transparent volume in the plot represents the 95% of rotational space where hydrogen bonding is allowed for steric reasons. Figure 6: DFT calculations for CH3–NH–CO–-CH3 dimer and CH3–NH–CO–CH2–NH–CO–CH3. ( a ) For each sampled point in rotational space, a sphere is plotted whose radius is proportional to the Boltzmann weight factor exp(−E/kT) of that point at room temperature with the normalization constant chosen such that points with 0.1 eV above the global minimum of −0.30 eV vanish. By this procedure, hydrogen bonds of at least 0.2 eV strength appear coloured in the figure and are found to comprise 32% of the entire volume of rotational space. Assessing the volume taken up by hydrogen bonds of at least 0.1 eV strength, one reaches 50% of the volume of rotational space.The most stable bonding class is that of the acceptor molecule binding through the O-lone pair, which is at the methyl side of the carbonyl (red spheres in the figure). The other significant bonding class is that of the acceptor molecule binding through the O-lone pair, which is at the amide side of the carbonyl (blue spheres in the figure). Both are doubly degenerate because of symmetry. ( b ) This plot is prepared just as ( a ) is, but here for two consecutive peptide units along the backbone, and only one bonding class (modulo symmetry) is identified. These two minima are recognized as γ + and γ − turns, respectively. ( c ) Plot of the volume in rotational space (black points) with prohibitive steric overlap of rigid atomic spheres. The transparent volume in the plot represents the 95% of rotational space where hydrogen bonding is allowed for steric reasons. Full size image Local hydrogen bond energy landscapes To probe the (non)-locality of the formation of the clusters in rotational space, we modelled hydrogen bonds between backbone peptide units by Density Function Theory (DFT), which has proven to be successful in describing basic secondary structure motifs [18] , [19] . We first probe the energy landscape of rotational space by modelling two peptide units as described under Methods. The resulting energy landscape ( Fig. 6a ), which in this case is twofold symmetric, describes, to some extend, the same overall part of rotational space as the experimental PDB based clustering shown in ( Fig. 1b–d ). Because of symmetry, the global minimum appears twice in rotational space. Two bonding classes are defined by which the O-lone pair is used (the methyl-side or the nitrogen side of the carbonyl) ( Fig. 6a ). The two classes of hydrogen bonding between two N -methylacetamide molecules span two large volumes of rotational space, meaning that the bonding is rather insensitive to the relative rotation of the two molecules; intrinsic properties of the hydrogen bond define the overall volume of spatial rotations. However, we must conclude that the fine clustering, which our analysis of PDB results in, does not arise from two free isolated peptide units, interacting in a single hydrogen bond. This strongly highlights the non-locality and importance of this observed clustering of rotations across hydrogen bonds in protein structures. Next we analyzed the influence of local backbone constraints on the energy landscape by modelling two fused methylacetamide molecules, which further interacts via an hydrogen bond from the one peptide unit to the immediate next one along the backbone (only possible with this short backbone). The configurations were relaxed as discussed under Methods, but the spanning of rotational space was limited to situations in which the length of the hydrogen bond was initially smaller than 3.5 Å; this excludes fully extended structures, which were also not included in our analysis of the PDB. The resulting energy landscape ( Fig. 6b ) shows two minima corresponding to γ + and γ − turns, which correspond to cluster and , respectively ( Fig. 5a ). The energy minima are now relatively weaker, which demonstrates the compromise between covalent backbone bonding and hydrogen bonds, where the high force constants of the covalent bonds present between the two C–C–N units drastically reduce the accessible configurations. This result together with the finding of a widespread minimum of the hydrogen bond in general ( Fig. 6a ) is strongly suggestive that the clusters empirically observed in protein structures are in part caused by geometric implications of the polypeptide backbone structure of the protein together with the identity of the residues, that is, the protein primary structure. Our rotational descriptor of main chain hydrogen bonds has been demonstrated to be an effective coordinate on the possible local geometries around hydrogen bonds and the geodesic distance in rotation space a useful measure of the discrepancy between two hydrogen bonds. The descriptor provides a uniform viewpoint on local configurations of peptide units participating in an hydrogen bond encompassing secondary structures and turns, and it displays a remarkable clustering over all hydrogen bonds in the PDB. Akin to Ramachandran plots, 3D plots in rotational space usefully depict the relative positions of peptide units across hydrogen bonds relevant for studying protein conformation, dynamics and pathways. Our overall hydrogen bond patterns could be used to annotate protein secondary and tertiary structure, which may lead to a valuable and robust new classification of protein folds [11] , [20] . NMR is a widely used technique for determining structures of proteins in solution [21] where it is common practice to calculate an ensemble of structures. The scatter within this ensemble derives from both genuine dynamics of the protein in solution and from lack of experimental constraints. Traditionally, this scatter is viewed by superimposing the structures and measuring coordinate differences [22] . However, this can be cumbersome and even misleading if large unstructured regions are present that mask more important structural features, for example, a dynamical hinge connecting two rigid regions. Our classification is a powerful tool for analyzing structural ensembles derived by X-ray/NMR, as visualization of rotations highlights important structural features while unstructured regions are omitted, for example, our method pinpoints only the dynamical part of a hinge. X-ray crystallography can yield very accurate structures, which are modelled to fit the observed electron-density maps. These maps, that integrate all available diffraction data, may contain less ordered local regions, and the quality of derived structures is overall limited by the resolution of the diffraction data and the accuracy of the determined phases. Among a number of validation tools and procedures to ensure model quality is the unbiased Ramachandran plot. Entirely analogously, our new constraints on hydrogen bond rotations provide hydrogen bond plot quality as a new tool to have a complementary role in model validation and refinement, especially in cases where phi–psi angle restraints defer any use of Ramachandran plot validation such as low-resolution crystallography, electron microscopy and in silico modelling. The further geometrically possible beta strands, we find here, comprised of clusters L c , L e and L f perhaps pose an interesting opportunity in de novo protein-structure design. As demonstrated [23] for RNA, free energies coupled to the topology of fatgraphs [8] labelled by nucleic acids can be effectively used to predict RNA secondary structure. Hydrogen bond free energy [5] , [24] relying on the distribution of hydrogen bond rotations within each cluster could be readily implemented as Boltzmann statistics based on HQ60 for example. Coupled to chord diagrams with chords labelled by cluster and the backbone labelled by amino acids, this could provide a new tool for ab initio protein folding. As rotations can be assigned to any ordered pair of peptide units, relationships between them beyond hydrogen bonding, such as spatial proximity, can be likewise studied. Suitable triples of vectors can moreover be similarly assigned to any oriented covalent bond and rotations used to study relationships between them. Our basic method could therefore be much more broadly applied to include protein side-chains or general ligands for example. A web-based implementation of our descriptor for uploaded PDB files is anonymously available at http://bion-server.au.dk/hbonds/ . Peptide plane rotation Associate a triple of three-dimensional vectors to the peptide unit P i of a protein containing the consecutive backbone atoms in the usual crystallographic notation as follows: In standard vector notation, where , , are the respective coordinates of , C i ,N i +1 . Such a triple is described by a 3-by-3 matrix the respective columns of which are the coordinates of , , in the standard vector basis. For any two peptide units P i and P j , with corresponding matrices and , the rotation brings to . However, this rotation will change if we rotate the entire protein. A descriptor, which is independent of overall rotation is obtained on transforming both of and by . Thus, becomes the standard vector basis and becomes . We use as our descriptor for the rotation bringing P i to P j . For three peptide units P i , P j , P k , we have the relation . In the special case when the two peptide units P i−1 and P i are consecutive along the backbone sharing the carbon , the rotation matrix is a function of the backbone conformational angle ϕ i preceding and ψ i following . Assuming the idealized geometry of exact tetrahedral angles among bonds at each alpha carbon atom and 120-degree angle between bonds within a peptide unit, one finds [8] , where, with C 1 =cos ϕ and S 1 =sin ϕ , and, with and , When peptide unit P i −1 is in cis conformation, the matrix must be premultiplied by a diagonal matrix with entries (1,−1,−1). Supplementary Table 3 lists the conformational angles defining the secondary structures considered in this paper from which the idealized backbone transition is calculated. Rotations and angle-axis pairs Let , , be the usual vector basis of space. A rotation must necessarily map these vectors to another respective triple of pairwise perpendicular vectors of length one with cross-product . We may write , for each r =1, 2, 3, to determine the matrix where the respective columns are the coordinates of . The trace of is the sum of its diagonal entries. One can compute the matrix corresponding to a given angle-axis pair as follows. First, associate to the matrix Ω with rows (0, − w , v )), ( w , 0, − u ) and (− v , u , 0), and finally define , where I denotes the 3-by-3 identity matrix, and Ω 2 =ΩΩ denotes the matrix product. Conversely, the angle-axis pair corresponding to the matrix is given by , 0≤ θ ≤π with , the vector of unit length proportional to ( a 32 − a 23 , a 13 − a 31 , a 21 − a 12 ) for the case 0< θ <π. When θ =0, the matrix A is the identity matrix and is undetermined. When θ =π, the axis is determined up to its sign only by the equations u 2 −1= a 11 , v 2 −1= a 22 , w 2 −1= a 33 , 2 uv = a 12 , 2 uw = a 13 and 2 vw = a 23 . To describe distances between the modes of the clusters and known secondary structures, it is useful to define the transpose to be the matrix derived from by interchanging rows and columns. The geodesic distance on rotational space between two rotations is determined by the angle in the angle-axis pair associated to the rotation , that is, the distance between and is Hence distances in rotational space are between 0 and π. A special property is bi-invariance in the sense that for any four rotations , that is, the distance is unchanged under matrix multiplication on both the right and left sides. Furthermore, one can show that the bi-invariant (un-normalized Haar) measure on the collection of rotations is given by , where in the coordinates ( x , y , z ) of our plots with total volume of rotational space equal to 8π 2 . Thus, densities of points in our plots must be appropriately scaled, and distances between rotations must be computed using . In particular, this means that a true evenly distribution on rotation space will in our presentation also result in an evenly distributed density. The clustering algorithm To perform the clustering (see Supplementary Note 3 for choice of clustering algorithm) of the rotations, it is convenient to transform all data points in rotational space by left multiplication with an element in rotational space to move most of the observed rotations away from the boundary sphere. The convenient rotation is given by 2.479, (−0.282, 0.907, −0.313) in angle-axis notation, which is a point of density with angle coordinate fairly close to π . Next, the cube (− π , π ) 3 is divided into 81 × 81 × 81 small ‘boxes’ with side lengths δ =2π/81, so box ( n , m , p ) has center ( x n , y m , z p ) with x n =− π +( n −0.5) δ and y m and z p defined similarly. Let n nmp denote the number of transformed data points within the box ( n , m , p ) if it lies entirely within the ball B of radius π. For a box B at the boundary of the sphere of radius π, we count the number of points in B as well as the neighbouring antipodal box. The density in a box is given by , where . To form the clusters, the algorithm first finds seeds for the clusters after the boxes have been ordered according to density. A box with a local maximum of the density becomes a seed if the P -value for testing equal rates in boxes with distance 1 and boxes with distance 2, to the box under consideration, is below 0.003, and the P -value for the similar test using boxes with distances 2 and 3 is below 0.01 (for the robustness of these conditions please see Supplementary Fig. 7 ). To make the procedure robust to the number of boxes used to divide (− π , π ) 3 and to enhance the possibility of finding clusters in low-density regions, a similar run is made with a 64 × 64 × 64 division. If two nearby seeds from the first run are joined only one is kept as a final seed, and if a new seed is found, new meaning that it is sufficiently apart from the seeds of the first round, this is included as a seed in the 81 × 81 × 81 division (see Supplementary Note 4 for a comparison of clusterings for varying box sizes). The method used corresponds to testing for a known probability of success in a binomial distribution. A large P -value indicates that there is not much difference between boxes with distance 1 and boxes with distance 2 (or boxes with distance 2 and boxes with distance 3), that is, the density is fairly flat, not pointing to a well-defined cluster mode, hence the test. A small P -value on the other hand points to a cluster with a well-defined mode point. Having established the seeds, the densities d nmp for varying n , m , p are ordered according to decreasing size. The algorithm adds one box at a time, where each added box becomes a member of a cluster if the box distance from the point to the cluster is one or two; if there are several competing clusters to join, we choose the one with the highest density for the box closest to the new point. Having run through all nonempty boxes, a second run is made to allow unclassified boxes from the first run to join nearby clusters when the rotational space distance is <1.5 times the width of a box. Except for the minor clusters , , , , , , , L e and L d , both of the P -values used to define a seed of a cluster are <10 −5 ( Supplementary Fig. 7 ). Hydrogen bond rotations in turns and helixes The hydrogen bond rotation between peptide units i and j can be calculated from the transformations along the backbone. Specifically ( Fig. 2 ), if the donor peptide unit is after the acceptor unit along the backbone, then i > j and the hydrogen bond rotation is if the donor peptide unit is before the acceptor unit along the backbone, then i < j and the hydrogen bond rotation is To correlate various clusters in rotational space with known structural motives, we use the rotations given by the formulae (6), (7) and (8) for as functions of conformational angles and the known conformational angles for various local loops, turns and helix structures ( Supplementary Table 3 ). For gamma turns, the hydrogen bond rotations are respectively, where and are the backbone transformations defined from the set of conformational angles listed in Supplementary Table 3 . For beta turns, the hydrogen bonds rotations are where T is the turn type, and the backbone rotations are derived from two sets of conformational angles listed in Supplementary Table 3 . For 3 10 , α and π helices, the hydrogen bond rotations are respectively, where , and are the respective backbone rotations. Supplementary Table 3 gives a complete list of the hydrogen bond rotations for all the considered secondary structures and turns assuming idealized geometry and exact cis or trans conformation. Hydrogen bond rotations in long-range clusters For the long-range clusters, we consider their association with ideal parallel or antiparallel beta strands. For an antiparallel beta strand, if there is an hydrogen bond between residue i and j with rotation , the next hydrogen bond further away from the loop has a rotation given by either or again under the assumption of ideal conformational angles along the backbone. For an extended antiparallel beta strand, we require . The corresponding relations for an ideal parallel beta strand are where is the ideal transformation along the backbone given in Supplementary Table 6 . See Supplementary Fig. 8 for an explanation of these relations. For the extended parallel case, we require . If , then we also have , and the only solutions are and a half–full turn around the axis of , the latter not being relevant for a parallel beta strand. If the conformational angles between the two hydrogen bonds correspond to an ideal antiparallel beta strand, then we can calculate the rotation of the next hydrogen bond from the rotation of the inner hydrogen bond by equation (15), where is the ideal transformation along the backbone. Next, consider the situation where the inner hydrogen bond of the loop belongs to one of the + clusters (2:4 hairpin). In this case, the next hydrogen bond belongs to the long-range clusters. Still assuming that the conformational angles between the two hydrogen bonds correspond to an ideal antiparallel beta strand, we get equation (16) instead of equation (15). We have probed for the existence of pairs and subject to either (15) or (16) as follows. For each turn cluster, we find candidate ’s as those hydrogen bonds with conformational angles outwards of the turn close to the ideal antiparallel conformational angles (−135°, 150°) allowing for a deviation of 30°. From the selected cases, we calculate an average hydrogen bond rotation , find from the above equations (15) and (16), and look for this rotation in the appropriate length category of hydrogen bonds. Density function theory DFT has been used to investigate the nature of the hydrogen bonds between backbone peptide units. The calculations were done using the ASE/GPAW package [25] using projector augmented waves and a real space basis (periodic boundary conditions in a 19.2 × 19.2 × 19.2 Å super cell and a grid-spacing of 0.16 Å). Exchange-correlation effects were described using the Perdew-Burke-Ernzerhof (PBE) functional. This functional has been proven successful in describing the hydrogen binding within, for example, helical polypeptides (including the transitions from the alpha-helix to the pi- and 3–10 helices) [18] and in describing the side-group propensities within beta-sheets [19] . We probe the entire energy landscape of rotational space by modelling two peptide units, minimalistically represented by methylacetamide, CH 3 –NH–CO–CH 3 . The relative position of the donor and acceptor is calculated for each position of rotational space followed by relaxation of all atomic degrees of freedom (except for the C–C–N coordinates, whose relative position are fixed and only allowed to translate as a rigid unit, so as to not change the rotation from one unit to the other). How to cite this article : Penner, R.C. et al . Hydrogen bond rotations as a uniform structural tool for analyzing protein architecture. Nat. Commun. 5:5803 doi: 10.1038/ncomms6803 (2014).